Lkb1 maintains Tregcell lineage identity Regulatory T (T reg ) cells are a distinct T-cell lineage characterized by sustained Foxp3 expression and potent suppressor function, but the upstream dominant factors that preserve T reg lineage-specific features are mostly unknown. Here, we show that Lkb1 maintains T reg cell lineage identity by stabilizing Foxp3 expression and enforcing suppressor function. Upon T-cell receptor (TCR) stimulation Lkb1 protein expression is upregulated in T reg cells but not in conventional T cells. Mice with T reg cell-specific deletion of Lkb1 develop a fatal early-onset autoimmune disease, with no Foxp3 expression in most T reg cells. Lkb1 stabilizes Foxp3 expression by preventing STAT4-mediated methylation of the conserved noncoding sequence 2 (CNS2) in the Foxp3 locus. Independent of maintaining Foxp3 expression, Lkb1 programs the expression of a wide spectrum of immunosuppressive genes, through mechanisms involving the augmentation of TGF-β signalling. These findings identify a critical function of Lkb1 in maintaining T reg cell lineage identity. Regulatory T (T reg ) cells preserve immune homeostasis by suppressing autoreactive immune responses [1] , [2] . The T reg cell lineage can be defined by two basic characteristics, stable expression of the transcription factor Foxp3 (forkhead box P3) and potent suppressive capacity [3] , [4] . T reg cells are stable and usually retain lineage characteristics in vivo [5] , [6] . However, under some conditions, T reg cells can lose or alter their lineage identity, resulting in immune disturbance and development of diseases [3] , [4] , [6] , [7] . Thus, delineating the molecular mechanisms that maintain the T reg lineage identity is important for understanding and treating T reg cell-related immune diseases. Foxp3 is the most specific marker for distinguishing T reg cells from other T cells and an important regulator required for programming T reg suppressive function [1] , [2] . Lineage tracing in mice has shown that thymus-derived mature T reg cells have relatively stable Foxp3 expression in both homeostasis and inflammatory conditions [5] . Other reports indicate that epigenetic demethylation of the conserved noncoding sequence 2 (CNS2, also known as T reg cell-specific demethylation region) in the Foxp3 locus can ensure stable Foxp3 expression in T reg cells [8] , [9] , [10] . However, the upstream signalling checkpoints that activate chromatin, and the demethylation status, of Foxp3 locus are not clear. T reg cells suppress immune responses through diverse mechanisms, such as the modulation of antigen presentation function (via CTLA4 (cytotoxic T-lymphocyte associated protein 4)), the production of inhibitory cytokines (for example, interleukin (IL)-10 and IL-35) and metabolites (for example, reactive oxygen species and adenosine), the deprivation of the T-cell growth factor IL-2 (via CD25), and the direct killing of target cells (via granzyme B and perforin) [2] , [11] , [12] . Although Foxp3 has an important function in programming T reg cells by controlling the expression of a large number of immunosuppressive genes, Foxp3 alone is not sufficient to confer this function [1] , [2] . In addition, T-cell receptor (TCR) signalling is also important to promote T reg cell function [13] , [14] , [15] . Nevertheless, little is known about other upstream ‘master regulators’ that broadly control the expression of these T reg cell-associated immunosuppressive genes. Liver kinase b1 (Lkb1) is a tumour suppressor, and is mutated in Peutz–Jeghers cancer syndrome, cervical carcinoma and many sporadic non-small-lung carcinomas [16] , [17] , [18] . Under energy-stressed conditions, Lkb1 is an important upstream kinase that phosphorylates AMP-activated protein kinase (AMPK) and AMPK-related kinases that coordinate cell growth with metabolism [16] , [17] , [18] . Lkb1 has been shown to restrain the activation and proinflammatory function of conventional T cells [18] , [19] . In this study, we find that Lkb1 protein is specifically increased in T reg cells upon TCR stimulation. To understand the function and mechanism of Lkb1 in T reg cells, we generate a mouse line with Lkb1 specifically deleted in T reg cells. These mice develop a fatal early-onset autoimmune disease with defective maintenance of stable Foxp3 expression and suppressive capacity in T reg cells. Mechanistically, Lkb1 restrains STAT4 (signal transducer and activator of transcription 4) activation partially through suppressing nuclear factor-κB (NF-κB) signalling, and thus prevents STAT4-mediated methylation of CNS2 in the Foxp3 locus, resulting in stable Foxp3 expression. Meanwhile, Lkb1 promotes the expression of a large number of immunosuppressive genes partially through augmenting transforming growth factor-β (TGF-β) signalling. Our study identifies Lkb1 as a critical determinant of T reg cell linage identity. Lkb1 protein is increased in T reg cells upon TCR stimulation TCR stimulation is essential for T reg cells to exert their optimal function [13] , [14] , [15] . Lkb1 protein expression in T reg cells were slightly lower compared with conventional T cells without stimulation ( Fig. 1a and Supplementary Figs 1a and 8a,b ). However, upon TCR stimulation, Lkb1 protein expression was markedly upregulated in T reg but not conventional T cells ( Fig. 1a and Supplementary Fig. 1a ), implying that Lkb1 might be particularly important for T reg cells to execute their immunoregulatory effect. 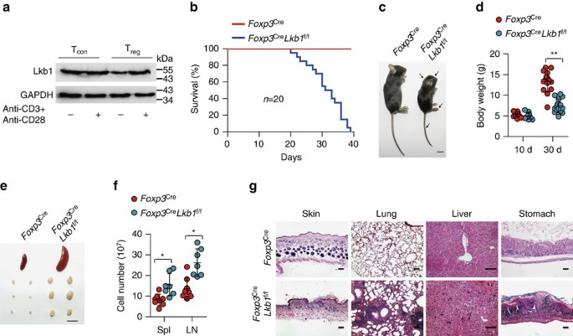Figure 1: Tregcell-specific deletion of Lkb1 leads to a fatal autoimmune disease. (a) Lkb1 proteins in CD4+YFP−conventional T cells and CD4+YFP+Tregcells untreated or stimulated in plates coated with anti-CD3 and anti-CD28 in the presence of IL-2 for 24 h determined by western blot. (b) Survival ofFoxp3CreandFoxp3CreLkb1f/fmice (n=20). (c) A representative appearance of 30-day-oldFoxp3CreandFoxp3CreLkb1f/fmice (scale bar, 1 cm). (d) Body weight ofFoxp3CreandFoxp3CreLkb1f/fmale mice of different ages (n=10–15). (e) A representative picture of spleen and lymph nodes from 30-day-oldFoxp3CreandFoxp3CreLkb1f/fmice. (scale bar, 1 cm). (f) Total cell numbers in spleen (Spl) and lymph nodes (LNs) ofFoxp3CreandFoxp3CreLkb1f/fmice (n=7–8). (g) Representative haematoxylin and eosin-stained skin, lung, liver and stomach sections fromFoxp3CreandFoxp3CreLkb1f/fmice (scale bar, 100 μm). All mice analysed were 28–30 days old, unless otherwise specified. Log-rank survival curve was used for survival analysis inb, and two-way analysis of variance (ANOVA) was used for statistical analyses ind,f(*P<0.05, **P<0.01, ****P<0.0001); error bars represent s.d.; all data are representative of at least three independent experiments. Figure 1: T reg cell-specific deletion of Lkb1 leads to a fatal autoimmune disease. ( a ) Lkb1 proteins in CD4 + YFP − conventional T cells and CD4 + YFP + T reg cells untreated or stimulated in plates coated with anti-CD3 and anti-CD28 in the presence of IL-2 for 24 h determined by western blot. ( b ) Survival of Foxp3 Cre and Foxp3 Cre Lkb1 f/f mice ( n =20). ( c ) A representative appearance of 30-day-old Foxp3 Cre and Foxp3 Cre Lkb1 f/f mice (scale bar, 1 cm). ( d ) Body weight of Foxp3 Cre and Foxp3 Cre Lkb1 f/f male mice of different ages ( n =10–15). ( e ) A representative picture of spleen and lymph nodes from 30-day-old Foxp3 Cre and Foxp3 Cre Lkb1 f/f mice. (scale bar, 1 cm). ( f ) Total cell numbers in spleen (Spl) and lymph nodes (LNs) of Foxp3 Cre and Foxp3 Cre Lkb1 f/f mice ( n =7–8). ( g ) Representative haematoxylin and eosin-stained skin, lung, liver and stomach sections from Foxp3 Cre and Foxp3 Cre Lkb1 f/f mice (scale bar, 100 μm). All mice analysed were 28–30 days old, unless otherwise specified. Log-rank survival curve was used for survival analysis in b , and two-way analysis of variance (ANOVA) was used for statistical analyses in d , f (* P <0.05, ** P <0.01, **** P <0.0001); error bars represent s.d. ; all data are representative of at least three independent experiments. Full size image Deletion of Lkb1 in T reg cells leads to a fatal autoimmunity To investigate the role of Lkb1 in T reg cells, we generated a mouse line with Lkb1 conditionally depleted in T reg cells by crossing Foxp3 YFP-Cre ( Foxp3 Cre , which ensure T reg cell-specific deletion of a target gene) mice [20] with Lkb1 f/f mice [21] . Lkb1 protein was depleted in CD4 + YFP + T reg cells from Foxp3 Cre Lkb1 f/f mice ( Supplementary Figs 1b and 8c,d ). Strikingly, loss of Lkb1 in T reg cells caused early moribund at ∼ 35 days of age ( Fig. 1b ). Foxp3 Cre Lkb1 f/f mice exhibited smaller size, decreased mobility, hunched posture, collapsed ears and tail skin lesions ( Fig. 1c ), and barely increased in body weight with age ( Fig. 1d ). Foxp3 Cre Lkb1 f/f mice displayed splenomegaly and lymphadenopathy ( Fig. 1e ), and they had increased cell numbers in secondary lymphoid organs ( Fig. 1f ). Histopathological analysis revealed massive infiltration of lymphocytes into multiple organs such as skin, lung, liver and stomach ( Fig. 1g ), suggesting T-cell autoimmunity. In support of this, Foxp3 Cre Lkb1 f/f mice had substantial expansion of CD4 + conventional T cells ( Supplementary Fig. 1c ), associated with drastically increased percentages of cells that displayed a CD44 high CD62L low effector/memory phenotype ( Fig. 2a and Supplementary Fig. 1d ). These mice also had higher percentages of CD4 + and CD8 + conventional T cells that expressed the proliferation marker Ki67 and acute activation markers CD25 and CD69 ( Fig. 2b and Supplementary Fig. 1e ), and produced the inflammatory cytokines interferon-γ, IL-4 and IL-17A ( Fig. 2c and Supplementary Fig. 1f ). These phenotypes were similar in severity to those observed in mice deficient of Foxp3 (ref. 22 ) or depleted of T reg cells [23] , indicating a severe defect of immune suppression mediated by T reg cells. 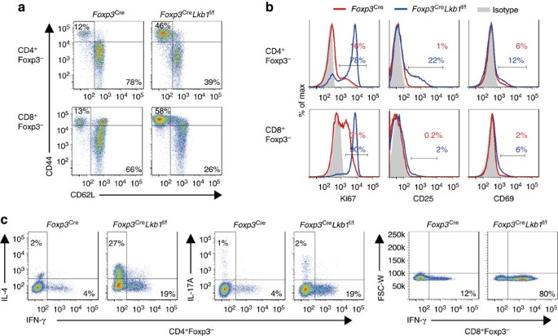Figure 2: Spontaneous activation of conventional T cells inFoxp3CreLkb1f/fmice. (a) Expression of CD44 and CD62L on splenic CD4+Foxp3−and CD8+Foxp3−T cells fromFoxp3CreandFoxp3CreLkb1f/fmice. (b) Expression of Ki67, CD25 and CD69 in splenic CD4+Foxp3−and CD8+Foxp3−T cells fromFoxp3CreandFoxp3CreLkb1f/fmice. (c) Intracellular staining of cytokines in splenic CD4+Foxp3−and CD8+Foxp3−T cells fromFoxp3CreandFoxp3CreLkb1f/fmice stimulated with phorbol myristate acetate (PMA) and ionomycin for 4 h. All mice analysed were 28–30 days old. All data are representative of at least three independent experiments. Figure 2: Spontaneous activation of conventional T cells in Foxp3 Cre Lkb1 f/f mice. ( a ) Expression of CD44 and CD62L on splenic CD4 + Foxp3 − and CD8 + Foxp3 − T cells from Foxp3 Cre and Foxp3 Cre Lkb1 f/f mice. ( b ) Expression of Ki67, CD25 and CD69 in splenic CD4 + Foxp3 − and CD8 + Foxp3 − T cells from Foxp3 Cre and Foxp3 Cre Lkb1 f/f mice. ( c ) Intracellular staining of cytokines in splenic CD4 + Foxp3 − and CD8 + Foxp3 − T cells from Foxp3 Cre and Foxp3 Cre Lkb1 f/f mice stimulated with phorbol myristate acetate (PMA) and ionomycin for 4 h. All mice analysed were 28–30 days old. All data are representative of at least three independent experiments. Full size image Lkb1 maintains Foxp3 expression and CNS2 demethylation T reg cells normally stay at a relatively constant abundance within the CD4 + T-cell population, and expand concomitantly with effector/memory T cells to preserve immune homeostasis during inflammation [24] . Although not altered at early ages, the percentages of peripheral T reg cells among CD4 + T-cell populations continuously dropped to ∼ 3% by 4 weeks of age when the mice became moribund ( Fig. 3a ). Despite greatly increased numbers of effector/memory T cells in Foxp3 Cre Lkb1 f/f mice ( Supplementary Fig. 1d ), the absolute numbers of T reg cells were only comparable with those in wild-type mice ( Supplementary Fig. 1g ), suggesting that Lkb1-deficient T reg cells fail to accumulate concomitantly with effector/memory T cells in Foxp3 Cre Lkb1 f/f mice at later ages that might contribute to the autoimmunity in Foxp3 Cre Lkb1 f/f mice. 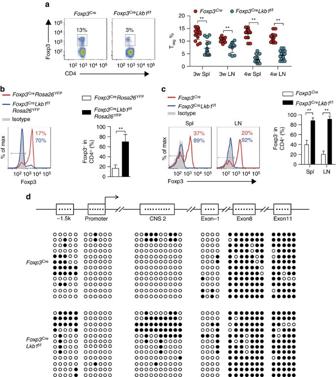Figure 3: Lkb1 stabilizesFoxp3expression and prevents CNS2 methylation. (a) Foxp3+cell percentages among CD4+T cells in spleen and lymph nodes fromFoxp3CreandFoxp3CreLkb1f/fmice of different ages (n=10–15). (b) Foxp3 expression in CD4+Rosa26-YFPhigh(Rosa26-YFP labelled the cells that have experienced the expression of Foxp3,Rosa26-YFP was much brighter than and thus distinguishable from Foxp3-YFP) cells fromFoxp3CreRosa26YFPandFoxp3CreLkb1f/fRosa26YFPmice. (c) Foxp3 expression in Tregcells doubly sorted fromFoxp3CreandFoxp3CreLkb1f/fmice and transferred together with Tncells intoRag1−/−mice for 3 weeks (n=3). (d) Methylation of the CpG motifs of the −1.5 kb region, promoter, CNS2, exon 1, exon 8 and exon 11 across theFoxp3locus in Tregcells fromFoxp3CreandFoxp3CreLkb1f/fmice, determined by bisulfite sequencing. Filled circles represent methylated CpG sites and open circles represent unmethylated CpG sites. Two-way analysis of variance (ANOVA) was used for statistical analyses ina,c, and unpaired two-tailed Student’st-test was used for statistical analyses inb(**P<0.01); error bars represent s.d.; all data are representative of at least two independent experiments. Figure 3: Lkb1 stabilizes Foxp3 expression and prevents CNS2 methylation. ( a ) Foxp3 + cell percentages among CD4 + T cells in spleen and lymph nodes from Foxp3 Cre and Foxp3 Cre Lkb1 f/f mice of different ages ( n =10–15). ( b ) Foxp3 expression in CD4 + Rosa26 -YFP high ( Rosa26 -YFP labelled the cells that have experienced the expression of Foxp3, Rosa26 -YFP was much brighter than and thus distinguishable from Foxp3-YFP) cells from Foxp3 Cre Rosa26 YFP and Foxp3 Cre Lkb1 f/f Rosa26 YFP mice. ( c ) Foxp3 expression in T reg cells doubly sorted from Foxp3 Cre and Foxp3 Cre Lkb1 f/f mice and transferred together with T n cells into Rag1 −/− mice for 3 weeks ( n =3). ( d ) Methylation of the CpG motifs of the −1.5 kb region, promoter, CNS2, exon 1, exon 8 and exon 11 across the Foxp3 locus in T reg cells from Foxp3 Cre and Foxp3 Cre Lkb1 f/f mice, determined by bisulfite sequencing. Filled circles represent methylated CpG sites and open circles represent unmethylated CpG sites. Two-way analysis of variance (ANOVA) was used for statistical analyses in a,c , and unpaired two-tailed Student’s t -test was used for statistical analyses in b (** P <0.01); error bars represent s.d. ; all data are representative of at least two independent experiments. Full size image The survival and proliferation of Lkb1-deficient T reg cells were barely altered compared with wild-type control cells ( Supplementary Fig. 2a,b ). Thus, other reasons might account for the defective accumulation of Lkb1-deficient T reg cells. T reg cells are considered a stable lineage marked by sustained Foxp3 expression [5] , but under certain conditions they might lose Foxp3 expression and develop into cells resembling effector T cells (designated ex-T reg cells) [25] . To investigate whether Lkb1-deficient T reg cells were prone to lose Foxp3 expression, we introduced the Rosa26 YFP allele (a loxp-site-flanked STOP cassette followed by the YFP-encoding sequence was inserted into the Rosa26 locus, and the expression of YFP from the Rosa26 locus was dependent on the expression of Cre recombinase) into wild-type and conditional knockout mice [26] . CD4 + Rosa26 -YFP high cells (100% Lkb1-deficient T reg cells) sorted from Foxp3 Cre Lkb1 f/f Rosa26 YFP mice contain much higher percentages of Foxp3 − cells (which represented ex-T reg cells that ever experienced Foxp3 expression but ceased to express it later) than that from Foxp3 Cre Rosa26 YFP mice ( Fig. 3b ). Therefore, a large proportion of Lkb1-deficient T reg cells lost Foxp3 expression and became ex-T reg cells that might result in the decrease of T reg cell abundance in vivo . Foxp3 is an X-chromosome-encoded transcription factor. Due to random X inactivation, female mice heterozygous for Foxp3 Cre ( Foxp3 Cre/+ ) should contain ∼ 1:1 ratio of Foxp3 Cre -positive T reg cells to Foxp3 Cre -negative T reg cells. Hence, the Foxp3 Cre -heterozygous female Foxp3 Cre/+ Lkb1 f/f mice were devoid of autoimmune diseases due to the presence of T reg cells lacking Foxp3 Cre expression but retaining a wild-type Lkb1 allele [8] . Proinflammatory cytokines may impair T reg cell stability [3] , [6] . To determine whether the instability of T reg cells was due to either the inflammatory environment in Foxp3 Cre Lkb1 f/f Rosa26 YFP mice or the intrinsic defect of the cells, we utilized Foxp3 Cre -heterozygous female Foxp3 Cre/+ Lkb1 f/f Rosa26 YFP mice that were devoid of autoimmune diseases. Despite the presence of wild-type T reg cells devoid of the expression of Foxp3 Cre in Foxp3 Cre/+ Lkb1 f/f Rosa26 YFP mice, the CD4 + Rosa26 -YFP high cells from these mice were cells that had ever experienced the expression of Foxp3 Cre that resulted in the deletion of Lkb1 and expression of Rosa26-YFP. Similarly, we observed substantially higher proportions of Foxp3 − cells among sorted CD4 + Rosa26 -YFP high cells from Foxp3 Cre/+ Lkb1 f/f Rosa26 YFP mice than that from Foxp3 Cre/+ Rosa26 YFP mice ( Supplementary Fig. 2c ), ruling out the possibility that overproduction of proinflammatory cytokines in Foxp3 Cre Lkb1 f/f mice were the causative reasons for T reg cell instability. Foxp3 − Rosa26 -YFP + ex-T reg cells might also arise from recently activated T cells that transiently expressed Foxp3 but did not develop into a full T reg program (which were also considered as poorly committed T reg cells) [27] . To determine whether the full committed T reg cells lose stability, we doubly sorted CD4 + CD25 + YFP + cells from CD45.1 + CD45.2 + wild-type Foxp3 Cre and CD45.1 − CD45.2 + Foxp3 Cre Lkb1 f/f mice, mixed them together with congenitally marked CD45.1 + CD45.2 − naive T (T n ) cells and transferred them into Rag1 −/− mice. Strikingly, we observed that nearly all the Lkb1-deficient T reg cells lost Foxp3 expression 3 weeks after transfer ( Fig. 3c ), despite the fact that most wild-type T reg cells retained Foxp3 expression. This was not due to the contamination of non-T reg cells because the starting population contained >99.5% Foxp3 + T reg cells after double sorting ( Supplementary Fig. 2d ). These results confirm that Foxp3 expression is lost in a large proportion of fully committed mature Lkb1-deficient T reg cells, rather than in a subset of poorly committed Foxp3 + cells. Next, we investigated the molecular mechanisms by which Lkb1 promoted T reg cell stability. Because Foxp3 protein expression level was barely altered in Lkb1-deficient T reg cells ( Supplementary Fig. 2e ), Lkb1 seemed to not control T reg stability through affecting Foxp3 protein production or degradation. The epigenetic status across the Foxp3 locus has been shown to be critical for sustained Foxp3 expression [9] . Two recent reports demonstrated that deletion of CNS2 region in the Foxp3 locus led to the loss of T reg cell stability [8] , [10] , suggesting that CNS2 is pivotal for maintaining stable Foxp3 expression in T reg cells. CNS2 is completely demethylated in T reg cells, but not in conventional T cells [9] , [28] , [29] , [30] . T reg cell lineage development is partially dependent on the demethylation of CNS2 (refs 31 , 32 ), and CNS2 has enhancer activity that is markedly reduced after methylation [31] . Therefore, we examined the methylation of CpG motifs across the Foxp3 locus by bisulfite sequencing in CD4 + YFP + T reg cells from Foxp3 Cre Lkb1 f/f mice and Foxp3 Cre mice, and found a significant increase (nearly 25%) in methylation of CpG at CNS2 in Lkb1-deficient T reg cells ex vivo ( Fig. 3d ). T reg cells that already lost Foxp3 expression were excluded in this analysis. Although Foxp3 promoter and other potentially regulatory regions are associated with T reg cell lineage identity [29] , [33] , [34] , the methylation of CpG at sites including −1.5 kb region, promoter, exon 1, exon 8 and exon 11 across the Foxp3 locus in Lkb1-deficient T reg cells was comparable to the wild-type T reg cells ( Fig. 3d ). Therefore, we hypothesize that methylation of CpG at CNS2 may contribute to the instability of Lkb1-deficient T reg cells. It seems that the methylation of CNS2 is not a secondary effect of Foxp3 reduction, because Foxp3 protein level was barely altered in Lkb1-deficient T reg cells that already had substantial CNS2 methylation. Given the critical role of CNS2 in conferring T reg cell stability established by previous studies, our results together suggested that CNS2 methylation might lead to the instability of Lkb1-deficient T reg cells. Lkb1 functions in T reg cells independent of AMPK AMPK is the well-known Lkb1 downstream target critical for coordinating metabolism [13] . Interestingly, we found no obvious decrease of AMPK activity in Lkb1-deficient Treg cells ( Supplementary Figs 3a and 8e–h ). Therefore, other kinases such as calmodulin-dependent protein kinase kinase-β (CamKKβ) and transforming growth factor-β-activated kinase-1 (TAK1) [15] may promote AMPK activation in T reg cells. These data argue that Lkb1 is not important for AMPK activation in T reg cells, and Lkb1 substrates other than AMPK are responsible for the observed phenotype of Lkb1-deficient T reg cells. Consistent with this, T reg cells that lacked the expression of AMPKα1/2 (from Foxp3 Cre AMPKα1 f/f AMPKα2 f/f mice, Supplementary Fig. 3b ) did not exhibit any adverse phenotype and in vivo functional impairment ( Supplementary Fig. 3c,d ). Lkb1 prevents STAT4 activation and STAT4 binding to CNS2 STAT3 and STAT6 are respectively the downstream mediators of the inflammatory cytokines IL-6 and IL-4 that bind to Foxp3 gene to mediate CpG methylation and T reg cell instability [8] , whereas the T reg cell growth factor IL-2 signals via STAT5 to counteract the destabilizing effect of these inflammatory cytokines [8] . Therefore, we examined whether the STAT family protein activations were altered in Lkb1-deficient T reg cells. Although STAT3 and STAT5 phosphorylations were barely affected, we detected a drastic increase of STAT4 phosphorylation and a slight increase of STAT6 phosphorylation in Lkb1-deficient T reg cells with or without the stimulation of relevant cytokines ( Fig. 4a and Supplementary Figs 4a,b and 8i–k ). The in vivo maintenance of T reg cells depends on their contact with dendritic cells (DCs) [35] , [36] , and hence we developed an in vitro DC-T reg cell co-culture system that could mimic the physiological situation to test which signalling would cause the instability of T reg cells. Lkb1-deficient T reg cells slightly lost stability when co-cultured with DCs without exogenous cytokines ( Fig. 4b ). Treatment with IL-2 alone, or IL-2 in combination with IL-4 or IL-6, did not lead to a significant loss of Foxp3 protein expression in Lkb1-deficient T reg cells after 4 days of culture ( Fig. 4c ). Strikingly, addition of IL-12, a potent STAT4 activator, caused the loss of Foxp3 expression in more than 50% Lkb1-deficient but not wild-type T reg cells ( Fig. 4c ), suggesting that STAT4 hyperactivation is the causative reason for the instability of Lkb1-deficient T reg cells. In addition, the apoptosis and proliferation were barely changed in Lkb1-deficient T reg cells compared with wild-type T reg cells ( Supplementary Fig. 4c,d ), suggesting that the loss of Foxp3 expressing Lkb1-deficient T reg cells in response to IL-2 + IL-12 is not due to their altered apoptosis or proliferation. Intriguingly, both divided and nondivided Lkb1-deficient T reg cells lost their stability ( Fig. 4d ). To determine whether the instability of Lkb1-deficient T reg cells was due to an intrinsic signalling alteration or in vivo selection of the T reg subpopulations with reduced stability, we used ERT2 Cre Lkb1 f/f Rosa26 YFP mice in which Lkb1 could be induced to be acutely deleted in T reg cells ( Supplementary Figs 4e and 8l,m ), thus avoiding the long-term in vivo selection. A similar IL-12-induced loss of stability was observed in T reg cells after induced Lkb1 deletion with 4-hydroxytamoxifen in vitro ( Fig. 4e ), implying an intrinsic role for STAT4 hyperactivation in destabilizing Lkb1-deficient T reg cells. 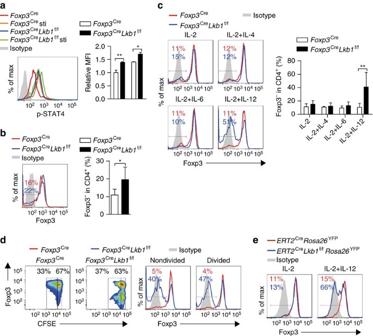Figure 4: Lkb1 prevents STAT4 activation to maintain Tregcell stability. (a) Intracellular phosphorylated STAT4 inFoxp3CreandFoxp3CreLkb1f/fTregcells treated with or without IL-12 (n=3). (b) Foxp3 expression inFoxp3CreandFoxp3CreLkb1f/fTregcells co-cultured with DCs without any cytokines (n=7). (c) Foxp3 expression inFoxp3CreandFoxp3CreLkb1f/fTregcells co-cultured with DCs supplemented with indicated cytokines (n=3). (d) Foxp3 expression in divided and nondividedFoxp3CreandFoxp3CreLkb1f/fTregcells co-cultured with DCs for 4 days supplemented with IL-2 and IL-12. (e) Foxp3 expression inERT2CreRosa26YFPandERT2CreLkb1f/fRosa26YFPTregcells co-cultured with DCs supplemented with indicated cytokines and 4-hydroxytamoxifen. Two-way analysis of variance (ANOVA) was used for statistical analyses ina,c, and unpaired two-tailed Student’st-test was used for statistical analyses inb(*P<0.05, **P<0.01); error bars represent s.d.; all data are representative of at least two independent experiments. Figure 4: Lkb1 prevents STAT4 activation to maintain T reg cell stability. ( a ) Intracellular phosphorylated STAT4 in Foxp3 Cre and Foxp3 Cre Lkb1 f/f T reg cells treated with or without IL-12 ( n =3). ( b ) Foxp3 expression in Foxp3 Cre and Foxp3 Cre Lkb1 f/f T reg cells co-cultured with DCs without any cytokines ( n =7). ( c ) Foxp3 expression in Foxp3 Cre and Foxp3 Cre Lkb1 f/f T reg cells co-cultured with DCs supplemented with indicated cytokines ( n =3). ( d ) Foxp3 expression in divided and nondivided Foxp3 Cre and Foxp3 Cre Lkb1 f/f T reg cells co-cultured with DCs for 4 days supplemented with IL-2 and IL-12. ( e ) Foxp3 expression in ERT2 Cre Rosa26 YFP and ERT2 Cre Lkb1 f/f Rosa26 YFP T reg cells co-cultured with DCs supplemented with indicated cytokines and 4-hydroxytamoxifen. Two-way analysis of variance (ANOVA) was used for statistical analyses in a , c , and unpaired two-tailed Student’s t -test was used for statistical analyses in b (* P <0.05, ** P <0.01); error bars represent s.d. ; all data are representative of at least two independent experiments. Full size image We then tested whether STAT4 could bind to and induce methylation of the Foxp3 locus in Lkb1-deficient T reg cells. Chromatin immunoprecipitation (ChIP) experiments showed that Lkb1-deficient T reg cells had significantly more STAT4 binding to the CNS2 than did the wild-type cells in response to IL-2 and IL-12 ( Fig. 5a and Supplementary Datas 1 and 2 ). Additionally, compared with IL-2 treatment alone, IL-2 and IL-12 treatment decreased STAT5 binding to the CNS2 in Lkb1-deficient T reg cells ( Fig. 5a ), suggesting that STAT4 might outcompete STAT5 in DNA binding in the Foxp3 locus. Since DNA methyltransferase (Dnmt) 1 and 3a were critical for maintaining and inducing DNA methylation respectively [37] , we tested whether STAT4 was capable of recruiting Dnmt1 or 3a to the Foxp3 locus. Lkb1-deficient T reg cells had significantly more Dnmt1 binding to the CNS2 than did the wild-type cells in response to IL-2 and IL-12 ( Fig. 5b ), consistent with the results of STAT4 ( Fig. 5a ). Notably, STAT4 associated with Dnmt1 but not Dnmt3a in T reg cells ( Fig. 5c and Supplementary Fig. 8n,o ). Furthermore, we examined the methylation of CNS2 in Foxp3 Cre and Foxp3 Cre Lkb1 f/f T reg cells treated with IL-2, IL-2+IL-12 or IL-2+IL-12+5-aza-deoxycytidine (5-aza-dC, a DNA methyltransferase inhibitor) to investigate the relationship between STAT4 and CNS2 methylation. In Foxp3 Cre Lkb1 f/f T reg cells, the methylation of CNS2 was higher after the treatment of IL-2+IL-12 compared with the treatment of IL-2 that could be reversed by 5-aza-dC ( Fig. 5d ). Indeed, the addition of 5-aza-dC rescued the loss of Foxp3 expression in Lkb1-deficient T reg cells ( Fig. 5e ). Since 5-aza-dC changes the global DNA methylation status, leading to the global changes in gene expression, we cannot exclude its effect on the expression of other genes. Nevertheless, these results together suggest that Lkb1 maintains stable Foxp3 expression in T reg cells under inflammatory conditions by preventing STAT4-mediated recruitment of Dnmt1 to and subsequent methylation of the Foxp3 CNS2. 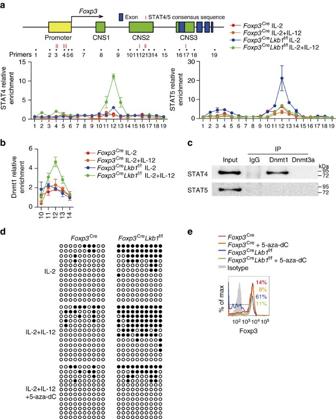Figure 5: Lkb1 prevents STAT4 binding to CNS2. (a) Binding of STAT4 and STAT5 to theFoxp3locus inFoxp3CreandFoxp3CreLkb1f/fTregcells treated with IL-2 or IL-2 plus IL-12, determined by ChIP. (b) Binding of Dnmt1 to the CNS2 ofFoxp3locus inFoxp3CreandFoxp3CreLkb1f/fTregcells treated with IL-2 or IL-2 plus IL-12, determined by ChIP. (c) STAT4 and STAT5 coprecipitation with Dnmt1 and Dnmt3a was analysed by using nuclear extract fromin vitroexpanded Tregcells. (d) Methylation of the CpG motifs of theFoxp3promoter and CNS2 inFoxp3CreandFoxp3CreLkb1f/fTregcells determined by bisulfite sequencing, and Tregcells were treated with indicated reagents. Filled circles represent methylated CpG sites and open circles represent unmethylated CpG sites. (e) Foxp3 expression inFoxp3CreandFoxp3CreLkb1f/fTregcells co-cultured with DCs supplemented with IL-2 plus IL-12 in the presence or absence of 5-aza-dC. All data are representative of at least two independent experiments. Figure 5: Lkb1 prevents STAT4 binding to CNS2. ( a ) Binding of STAT4 and STAT5 to the Foxp3 locus in Foxp3 Cre and Foxp3 Cre Lkb1 f/f T reg cells treated with IL-2 or IL-2 plus IL-12, determined by ChIP. ( b ) Binding of Dnmt1 to the CNS2 of Foxp3 locus in Foxp3 Cre and Foxp3 Cre Lkb1 f/f T reg cells treated with IL-2 or IL-2 plus IL-12, determined by ChIP. ( c ) STAT4 and STAT5 coprecipitation with Dnmt1 and Dnmt3a was analysed by using nuclear extract from in vitro expanded T reg cells. ( d ) Methylation of the CpG motifs of the Foxp3 promoter and CNS2 in Foxp3 Cre and Foxp3 Cre Lkb1 f/f T reg cells determined by bisulfite sequencing, and T reg cells were treated with indicated reagents. Filled circles represent methylated CpG sites and open circles represent unmethylated CpG sites. ( e ) Foxp3 expression in Foxp3 Cre and Foxp3 Cre Lkb1 f/f T reg cells co-cultured with DCs supplemented with IL-2 plus IL-12 in the presence or absence of 5-aza-dC. All data are representative of at least two independent experiments. Full size image Lkb1 restrains STAT4 and NF-κB signalling The Stat4 and Il12rb2 mRNA and IL-12Rβ2 protein expression levels were elevated in Lkb1-deficient T reg cells that could explain the increased STAT4 phosphorylation in these cells in response to IL-12 ( Supplementary Fig. 5a,b ). To determine which signalling promotes Stat4 and Il12rb2 expression in Lkb1-deficient T reg cells, we examined the activation of NF-κB and AKT, the major signalling mediators driving T helper type cell development [38] , [39] . We found that NF-κB p65 but not AKT was hyperactivated in Lkb1-deficient T reg cells ( Fig. 6a and Supplementary Figs 5c,d and 8p–r ), and the chemical inhibitors to NF-κB reduced Stat4 and Il12rb2 mRNA expression ( Fig. 6b ), as well as STAT4 phosphorylation ( Fig. 6c ). In addition, conserved NF-κB binding sites were present at the Stat4 and Il12rb2 loci ( Supplementary Data 1 ), and ChIP experiments demonstrated more binding of NF-κB p65 to Stat4 and Il12rb2 in Lkb1-deficient T reg cells than in wild-type cells ( Fig. 6d and Supplementary Datas 1 and 2 ), suggesting a direct role of NF-κB activation in promoting Stat4 and Il12rb2 transcription. Of note, chemical inhibitors of NF-κB could partially rescue the instability of Lkb1-deficient T reg cells ( Fig. 6e ). These results collectively indicate an involvement of NF-κB activation in driving STAT4 activation and instability of Lkb1-deficient T reg cells. 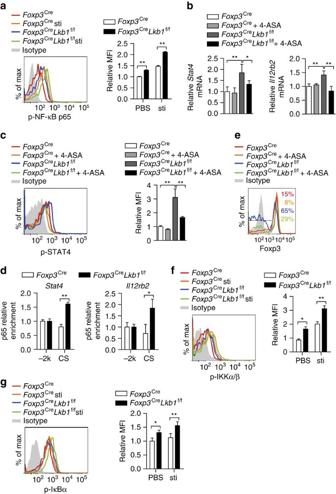Figure 6: Lkb1 suppresses NF-κB signalling to restrain STAT4 activation. (a) Intracellular phosphorylated NF-κB p65 inFoxp3CreandFoxp3CreLkb1f/fTregcells with or without IL-2 stimulation (n=3). (b)Stat4andIl12rb2mRNA inFoxp3CreandFoxp3CreLkb1f/fTregcells supplemented with or without 4-ASA for 16 h (n=3). (c) Intracellular phosphorylated STAT4 inFoxp3CreandFoxp3CreLkb1f/fTregcells supplemented with or without 4-ASA (n=3). (d) P65 enrichment to consensus sequences (CS) inStat4andIl12rb2locus inFoxp3CreandFoxp3CreLkb1f/fTregcells determined by ChIP. (e) Foxp3 expression inFoxp3CreandFoxp3CreLkb1f/fTregcells co-cultured with DCs supplemented with IL-2 and IL-12, with or without 4-ASA. (f) Intracellular phosphorylated IKKα (Ser176/180)/β (Ser177/181) inFoxp3CreandFoxp3CreLkb1f/fTregcells with or without IL-2 stimulation (n=3). (g) Intracellular phosphorylated IκBα (Ser 32/36) inFoxp3CreandFoxp3CreLkb1f/fTregcells with or without IL-2 stimulation (n=3). Two-way analysis of variance (ANOVA) was used for statistical analyses in (a,b,c,d,f,g) (*P<0.05, **P<0.01); error bars represent s.d.; all data are representative of at least two independent experiments. Figure 6: Lkb1 suppresses NF-κB signalling to restrain STAT4 activation. ( a ) Intracellular phosphorylated NF-κB p65 in Foxp3 Cre and Foxp3 Cre Lkb1 f/f T reg cells with or without IL-2 stimulation ( n =3). ( b ) Stat4 and Il12rb2 mRNA in Foxp3 Cre and Foxp3 Cre Lkb1 f/f T reg cells supplemented with or without 4-ASA for 16 h ( n =3). ( c ) Intracellular phosphorylated STAT4 in Foxp3 Cre and Foxp3 Cre Lkb1 f/f T reg cells supplemented with or without 4-ASA ( n =3). ( d ) P65 enrichment to consensus sequences (CS) in Stat4 and Il12rb2 locus in Foxp3 Cre and Foxp3 Cre Lkb1 f/f T reg cells determined by ChIP. ( e ) Foxp3 expression in Foxp3 Cre and Foxp3 Cre Lkb1 f/f T reg cells co-cultured with DCs supplemented with IL-2 and IL-12, with or without 4-ASA. ( f ) Intracellular phosphorylated IKKα (Ser176/180)/β (Ser177/181) in Foxp3 Cre and Foxp3 Cre Lkb1 f/f T reg cells with or without IL-2 stimulation ( n =3). ( g ) Intracellular phosphorylated IκBα (Ser 32/36) in Foxp3 Cre and Foxp3 Cre Lkb1 f/f T reg cells with or without IL-2 stimulation ( n =3). Two-way analysis of variance (ANOVA) was used for statistical analyses in ( a , b , c , d , f , g ) (* P <0.05, ** P <0.01); error bars represent s.d. ; all data are representative of at least two independent experiments. Full size image IκB (inhibitor of NF-κB) kinase (IKK) phosphorylates IκB, leading to their degradation and activation of transcription factor NF-κB. IKK is composed of three subunits, the similar protein kinases IKKα and IKKβ, and a regulatory subunit IKKγ [40] . The phosphorylations serines (Ser) in IKKα (Ser 176/180)/β (Ser 177/181) and IκBα (Ser 32/36) were all increased in Lkb1-deficient T reg cells ( Fig. 6f,g ), suggesting that Lkb1 might dampen NF-κB signalling by inhibiting IKKα/β activation. Lkb1 promotes the expression of immunosuppressive genes We further explored whether there are defects in Lkb1-deficient T reg cells that did not lose Foxp3 expression yet. The T-cell activation phenotype was already obvious ( Fig. 7a,b ) in 9–11-day-old Foxp3 Cre Lkb1 f/f mice that had normal percentages of T reg cells among CD4 + T cells ( Fig. 7c ), suggesting that the suppressor function of Lkb1-deficient T reg cells might be impaired. Indeed, in vitro T reg suppression assay showed that with different T reg to T n ratios, Lkb1-deficient T reg cells could not efficiently suppress the proliferation of responder T cells ( Fig. 7d ), indicating an impaired suppressive capacity of Lkb1-deficient T reg cells. 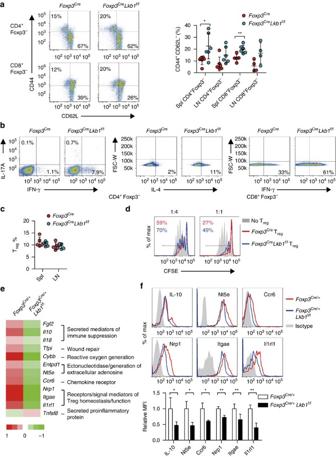Figure 7: Lkb1 promotes the expression of diverse immunosuppressive genes. (a) CD44highCD62Lloweffector/memory cells among splenic CD4+Foxp3−and CD8+Foxp3−T cells from 9–11-day-oldFoxp3CreandFoxp3CreLkb1f/fmice (n=4–6). (b) Intracellular staining of cytokines in splenic CD4+Foxp3−and CD8+Foxp3−T cells from 9–11-day-oldFoxp3CreandFoxp3CreLkb1f/fmice stimulated with phorbol myristate acetate (PMA) and ionomycin for 4 h. (c) Percentages of Foxp3+Tregcells among CD4+T cells in the spleen and lymph nodes from 9–11-day-oldFoxp3CreandFoxp3CreLkb1f/fmice (n=5). (d) Suppression of proliferation of CFSE-labelled Tncells (responding cells, Tresp) by different ratios of CD4+YFP+Tregcells fromFoxp3CreandFoxp3CreLkb1f/fmice. Trespcell division was determined by CFSE dilution at the indicated ratios of cell numbers between Tregcell and Trespcells. The experiment was repeated three times. (e) Tregcell function-related genes differentially expressed between CD4+YFP+Tregcells fromFoxp3Cre/+andFoxp3Cre/+Lkb1f/fmice determined by transcriptional profiling, shown in groups based on their functions. Fold difference means fold change of gene expression levels in Tregcells fromFoxp3CreLkb1f/fmice compared with that fromFoxp3Cremice. (f) Expression of indicated proteins on splenic Tregcells fromFoxp3Cre/+andFoxp3Cre/+Lkb1f/fmice (n=3). Two-way analysis of variance (ANOVA) was used for statistical analyses in (a,c,f) (*P<0.05, **P<0.01); error bars represent s.d.; all data are representative of at least two independent experiments. Figure 7: Lkb1 promotes the expression of diverse immunosuppressive genes. ( a ) CD44 high CD62L low effector/memory cells among splenic CD4 + Foxp3 − and CD8 + Foxp3 − T cells from 9–11-day-old Foxp3 Cre and Foxp3 Cre Lkb1 f/f mice ( n =4–6). ( b ) Intracellular staining of cytokines in splenic CD4 + Foxp3 − and CD8 + Foxp3 − T cells from 9–11-day-old Foxp3 Cre and Foxp3 Cre Lkb1 f/f mice stimulated with phorbol myristate acetate (PMA) and ionomycin for 4 h. ( c ) Percentages of Foxp3 + T reg cells among CD4 + T cells in the spleen and lymph nodes from 9–11-day-old Foxp3 Cre and Foxp3 Cre Lkb1 f/f mice ( n =5). ( d ) Suppression of proliferation of CFSE-labelled T n cells (responding cells, T resp ) by different ratios of CD4 + YFP + T reg cells from Foxp3 Cre and Foxp3 Cre Lkb1 f/f mice. T resp cell division was determined by CFSE dilution at the indicated ratios of cell numbers between T reg cell and T resp cells. The experiment was repeated three times. ( e ) T reg cell function-related genes differentially expressed between CD4 + YFP + T reg cells from Foxp3 Cre/+ and Foxp3 Cre/+ Lkb1 f/f mice determined by transcriptional profiling, shown in groups based on their functions. Fold difference means fold change of gene expression levels in T reg cells from Foxp3 Cre Lkb1 f/f mice compared with that from Foxp3 Cre mice. ( f ) Expression of indicated proteins on splenic T reg cells from Foxp3 Cre/+ and Foxp3 Cre/+ Lkb1 f/f mice ( n =3). Two-way analysis of variance (ANOVA) was used for statistical analyses in ( a , c , f ) (* P <0.05, ** P <0.01); error bars represent s.d. ; all data are representative of at least two independent experiments. Full size image To investigate the molecular mechanisms by which Lkb1 controls T reg cell function, we compared the transcriptional profiling of CD4 + YFP + T reg cells sorted from Foxp3 Cre/+ mice with that from Foxp3 Cre/+ Lkb1 f/f mice lacking autoimmune diseases, thus avoiding the secondary impact of the inflammatory environment on T reg cell gene expression ( Supplementary Data 3 ). Kyoto Encyclopedia of Genes and Genomes (KEGG) pathway analysis revealed that the most altered pathways were enriched for genes regulating immune function ( Supplementary Fig. 6a ). Intriguingly, Lkb1-deficient T reg cells have reduced expression of a wide variety of genes critically involved in T reg cell suppressor function including those encoding secreted molecules associated with immune suppression ( Fgl2 , Il10 and Il18 ) [11] , [41] , factors in wound-healing processes ( Tfpi ) [11] , regulators of reactive oxygen generation ( Cybb ) [11] , enzymes catalysing the generation of adenosine that directly inhibit proliferation of effector T cells ( Entpd1 and Nt5e ) [11] , [42] , chemokine receptors critical for T reg cell migration ( Ccr6 ) [43] and cell surface molecules facilitating T reg cell suppressor functions in either tumour environment ( Nrp1 ) [44] or organ-specific inflammatory conditions ( Itgae and Il1rl1 ) [45] , [46] ( Fig. 7e and Supplementary Fig. 6b ). On the other hand, the loss of Lkb1 promoted the expression of genes encoding proinflammatory mediators ( Tnfsf8 ) [11] ( Fig. 7e and Supplementary Fig. 6b ). It was further confirmed that Lkb1-deficient T reg cells from Foxp3 Cre/+ Lkb1 f/f mice had decreased protein levels of IL-10, Nt5e, Ccr6, Nrp1, Itgae and Il1rl1 ( Fig. 7f ). Most gene expression alterations were also recapitulated in T reg cells from Foxp3 Cre Lkb1 f/f mice ( Supplementary Fig. 6b ). These results clearly showed that Lkb1 promoted the immunosuppressive programs in T reg cells. TGF-β signalling in Lkb1-implemented T reg cell function TGF-β signalling plays crucial roles in T reg cell generation and function [47] . Transcriptional profiling analysis showed that Lkb1-deficient T reg cells express lower levels of Tgfbr1 and Tgfbr2 mRNA that was confirmed by real-time PCR and western blot ( Fig. 8a and Supplementary Figs 7a and 8s,t ). Hence, we proposed that this pathway might be defective in Lkb1-deficient T reg cells. Indeed, Smad2 (Ser 456/457)/Smad3 (Ser 423/425) phosphorylation was decreased ( Fig. 8b ), and Smad-DNA binding assay indicated that Smad transcriptional activity was impaired in Lkb1-deficient T reg cells ( Fig. 8c ). To determine whether impaired TGF-β signalling contributed to the impairment of Lkb1-deficient T reg cells, we conducted loss-of-function experiments by generating a mouse line with TGF-βR2 specifically deleted in T reg cells ( Foxp3 Cre Tgfbr2 f/f , Supplementary Figs 7b and 8u,v ) that displayed decreased Smad activation ( Supplementary Fig. 7c ). Although Foxp3 Cre Tgfbr2 f/f mice did not show overt autoimmune disease, increased percentages of CD44 high CD62L low effector/memory T cells ( Fig. 8d ) were observed despite a slightly increased T reg cell frequency among CD4 + T cells ( Fig. 8e ), indicating the functional impairment of TGF-βR2-deficient T reg cells. Consistently, TGF-βR2-deficient T reg cells displayed impaired suppressive capacity in vitro ( Fig. 8f ). To determine the global effects of defective TGF-β signalling on gene transcription, we conducted transcriptional profiling and found that TGF-βR2 deficiency led to the decreased expression of many genes important for T reg cell suppressor function ( Supplementary Data 4 ). Remarkably, TGF-βR2 deficiency recapitulated part of the suppressor gene expression alterations in Lkb1-deficient T reg cells, including Nt5e , Ccr6 , Nrp1 , Itgae and Il1rl1 ( Fig. 8g and Supplementary Data 4 ), that was also confirmed at protein levels ( Fig. 8h,i ). However, the Lkb1-regulated Fgl2 , Il10 , Tfpi , Entpd1 and Tnfsf8 transcripts were not altered in TGF-βR2-deficient T reg cells, suggesting that Lkb1 also utilize TGF-β-independent mechanisms to promote T reg cell function. To further determine whether lower expression of TGF-βR2 was the causative reason for impaired suppression function of Lkb1-deficient T reg cells, we generated T reg cells (from Foxp3 Cre and Foxp3 Cre Lkb1 f/f mice) transduced with retrovirus carrying TGF-βR2 complementary DNA (cDNA). TGF-βR2 was successfully expressed in RFP + YFP + T reg cells ( Supplementary Fig. 7c ). Overexpression of TGF-βR2 could partially rescue the expression of suppressor genes and suppression function of Lkb1-deficient T reg cells ( Fig. 8j and Supplementary Fig. 7d,e ). Together, these results indicate that Lkb1 implements T reg cell function partially through promoting TGF-β signalling. TGF-βR2-deficient T reg cells did not lose stability when co-transferred with T n cells into Rag1 −/− mice ( Fig. 8k ), suggesting that the decreased expression of TGF-β receptors does not account for the instability of Lkb1-deficient T reg cells. 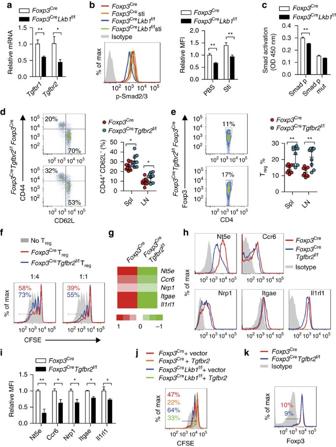Figure 8: TGF-β signalling is involved in Lkb1-implemented Tregcell suppressor function. (a)Tgfbr1andTgfbr2mRNA expression inFoxp3CreandFoxp3CreLkb1f/fTregcells by real-time PCR (n=3). (b) Intracellular expression of phosphorylated Smad2/3 in Tregcells fromFoxp3CreandFoxp3CreLkb1f/fmice, with or without TGF-β stimulation (n=3). (c) Binding capacity of Smad2/3 to recognized DNA sequences in nuclear lysates extracted from Tregcells fromFoxp3CreandFoxp3CreLkb1f/fmice. (d) CD44 and CD62L expression on CD4+Foxp3−T cells from 6-week-oldFoxp3CreandFoxp3CreTgfbr2f/fmice (n=6–11). (e) Foxp3 expression in CD4+T cells from 6-week-oldFoxp3CreandFoxp3CreTgfbr2f/fmice (n=6–11). (f) Suppression of proliferation of Tncells labelled with CFSE by different ratios of CD4+YFP+Tregcells fromFoxp3CreandFoxp3CreTgfbr2f/fmice. The experiment was repeated three times. (g) Some genes differentially expressed between CD4+YFP+Tregcells fromFoxp3CreandFoxp3CreTgfbr2f/fTregcells determined by transcriptional profiling. Fold difference means fold change of gene expression levels in Tregcells fromFoxp3CreTgfbr2f/fmice compared with that fromFoxp3Cremice. (h,i) Expression of indicated proteins on splenic Tregcells fromFoxp3CreandFoxp3CreTgfbr2f/fmice (n=3). (j) Suppression of proliferation of Tncells labelled with CFSE by different ratios of CD4+YFP+Tregcells fromFoxp3CreandFoxp3CreLkb1f/fmice that were transduced with retrovirus carrying TGF-βR2 or control vector. (k) Foxp3 expression in CD4+YFP+Tregcells doubly sorted fromFoxp3CreandFoxp3CreTgfbr2f/fmice and transferred together with Tncells intoRag1−/−mice for 3 weeks. Two-way analysis of variance (ANOVA) was used for statistical analyses in (a,b,c,d,e,i) (*P<0.05, **P<0.01); error bars represent s.d.; all data are representative of at least two independent experiments. Figure 8: TGF-β signalling is involved in Lkb1-implemented T reg cell suppressor function. ( a ) Tgfbr1 and Tgfbr2 mRNA expression in Foxp3 Cre and Foxp3 Cre Lkb1 f/f T reg cells by real-time PCR ( n =3). ( b ) Intracellular expression of phosphorylated Smad2/3 in T reg cells from Foxp3 Cre and Foxp3 Cre Lkb1 f/f mice, with or without TGF-β stimulation ( n =3). ( c ) Binding capacity of Smad2/3 to recognized DNA sequences in nuclear lysates extracted from T reg cells from Foxp3 Cre and Foxp3 Cre Lkb1 f/f mice. ( d ) CD44 and CD62L expression on CD4 + Foxp3 − T cells from 6-week-old Foxp3 Cre and Foxp3 Cre Tgfbr2 f/f mice ( n =6–11). ( e ) Foxp3 expression in CD4 + T cells from 6-week-old Foxp3 Cre and Foxp3 Cre Tgfbr2 f/f mice ( n =6–11). ( f ) Suppression of proliferation of T n cells labelled with CFSE by different ratios of CD4 + YFP + T reg cells from Foxp3 Cre and Foxp3 Cre Tgfbr2 f/f mice. The experiment was repeated three times. ( g ) Some genes differentially expressed between CD4 + YFP + T reg cells from Foxp3 Cre and Foxp3 Cre Tgfbr2 f/f T reg cells determined by transcriptional profiling. Fold difference means fold change of gene expression levels in T reg cells from Foxp3 Cre Tgfbr2 f/f mice compared with that from Foxp3 Cre mice. ( h , i ) Expression of indicated proteins on splenic T reg cells from Foxp3 Cre and Foxp3 Cre Tgfbr2 f/f mice ( n =3). ( j ) Suppression of proliferation of T n cells labelled with CFSE by different ratios of CD4 + YFP + T reg cells from Foxp3 Cre and Foxp3 Cre Lkb1 f/f mice that were transduced with retrovirus carrying TGF-βR2 or control vector. ( k ) Foxp3 expression in CD4 + YFP + T reg cells doubly sorted from Foxp3 Cre and Foxp3 Cre Tgfbr2 f/f mice and transferred together with T n cells into Rag1 −/− mice for 3 weeks. Two-way analysis of variance (ANOVA) was used for statistical analyses in ( a , b , c,d , e , i ) (* P <0.05, ** P <0.01); error bars represent s.d. ; all data are representative of at least two independent experiments. Full size image Here, we demonstrate that mice with T reg cell-specific deletion of Lkb1 develop a fatal, early-onset, autoimmune disease with moribund at ∼ 35 days of age. Such a fulminant disease is comparable to that observed in mice devoid of T reg cells or deficient in Foxp3 . Similar devastating diseases have also been reported to be present in mice with selective deficiency of Foxo1 (ref. 48 ) or Raptor, the rapamycin sensitive partner of mTORC1 (mammalian target of rapamycin complex 11) [26] in T reg cells, due to impaired T reg cell function. Intriguingly, Lkb1-deficient T reg cells lost their linage-specific features and exhibited severe impairment in the maintenance of Foxp3 expression and suppressor function that may underlie the extremely severe autoimmunity in Foxp3 Cre Lkb1 f/f mice. Although Lkb1 expression is not restricted to T reg cells, T reg cells substantially upregulate Lkb1 protein expression upon TCR stimulation. Given that TCR signalling is essential for T reg cell homeostasis and function, TCR-induced upregulation of Lkb1 protein may represent a critical feed-forward loop to stabilize T reg cell lineage identity. It is generally recognized that Foxp3 expression is highly stable in T reg cells. Whether a small proportion of T reg cells can lose Foxp3 expression in certain conditions is a controversial topic [6] . Some studies showed that T reg cells could lose Foxp3 expression and become ‘ex-T reg ’ cells under certain conditions [25] , while others argued that the so-called ‘ex-T reg ’ cells just might be the conventional T cells that transiently express Foxp3, namely poorly committed T reg cells [27] . Here, we showed that deficiency of Lkb1 caused very severe defects in T reg cell stability. More than 70% of T reg cells lost stability in Foxp3 Cre Lkb1 f/f Rosa26 YFP mice. In addition, the majority of the Lkb1-deficientT reg cells lost Foxp3 expression after being transferred into Rag1 −/− mice, indicating that Lkb1-deficient mature T reg cells continuously lost Foxp3 expression, rather than that a subset of Lkb1-deficient T cells only transiently expressed Foxp3 (poorly committed T reg cells). Such a severe defect was rarely reported in literatures, placing Lkb1 as a particularly important maintainer of Foxp3 stability. The demethylated status of Foxp3 CNS2 is critically involved in the maintenance of stable Foxp3 expression in T reg cells [8] , [9] , [10] , [28] , [29] , [30] , [31] , [32] . Substantial methylation of CNS2 but not promoter was observed in Lkb1-deficient T reg cells. Treatment of IL-12 further enhanced the methylation of CNS2 and caused the loss of Foxp3 expression in Lkb1-deficient but not wild-type T reg cells. Moreover, the DNA methyltransferase inhibitor 5-aza-dC reduced the methylation of CNS2 and rescued the instability of Lkb1-deficient T reg cells. These results suggest that Lkb1 stabilizes Foxp3 expression by building up the demethylated status of CNS2. It has been recently reported that deletion of CNS2 caused cell-division-dependent loss of Foxp3 expression [8] , [10] . In contrast, both divided and nondivided Lkb1-deficient T reg cells lost Foxp3 expression, suggesting that Lkb1 might also promote Foxp3 expression by CNS2-independent mechanisms, which need future exploration. The role of STAT4 in T reg cells is not well defined. Here we showed that deficiency of Lkb1 in T reg cells resulted in markedly more IL-12-induced STAT4 activation and STAT4 binding to CNS2. STAT4 associated with Dnmt1 and DNA methyltransferase chemical inhibitor rescued the instability of Lkb1-deficient T reg cells in response to IL-12. Thus, Lkb1 suppresses IL-12/STAT4 activation to stabilize Foxp3 expression in T reg cells. We further showed that NF-κB signalling is activated in Lkb1-deficient T reg cells, that increased Il12rb2 and Stat4 mRNA expression and STAT4 activation. However, inhibition of NF-κB signalling can only partially rescue the instability of Lkb1-deficient T reg cells, implicating that NF-κB-independent signalling mechanisms might also contribute to the unstable Foxp3 expression in Lkb1-deficient T reg cells. Independent of maintaining Foxp3 expression, Lkb1 also promotes T reg cell-suppressive capacity. Loss of Lkb1 in T reg cells results in the moderate downregulation of a number of immunosuppressive genes ( Fgl2 , Tfpi , Cybb , Entpd1 , Nt5e , Nrp1 , Itgae , Il18 , Il10 , Ccr6 , Il1rl1 ), suggesting that Lkb1 implements T reg cell function through broadly promoting T reg suppressor gene expression program. Lkb1 has been previously shown to positively or negatively regulate TGF-β/Smad signalling in a cell type-dependent manner [49] , [50] , but the precise mechanism is not fully elucidated. Here, we found the effect of Lkb1 on promoting T reg suppressor function was partially dependent on its augmentation of TGF-β signalling. TGF-β pathway is important for T reg cell development in the thymus and periphery [47] , [51] , [52] , but whether and how it affects T reg cell function remain poorly understood. Our results demonstrate that TGF-βR2-deficient T reg cells have impaired suppressive capacity associated with decreased expression of a number of genes associated with immune suppression ( Nt5e , Ccr6 , Nrp1 , Itgae and Il1rl1 ), partially recapturing the suppressor gene expression alterations in Lkb1-deficient T reg cells. Furthermore, overexpression of TGF-βR2 partially rescued the expression of certain suppressor genes and the suppressor function of Lkb1-deficient T reg cells, supporting that impaired TGF-β signalling contributed to the impaired suppressor function of Lkb1-deficient T reg cells. However, numerous Lkb1-regulated genes, including Fgl2 , Tfpi , Cybb , Entpd1 and Il18 , were not changed in TGF-βR2-deficient T reg cells, suggesting that TGF-β-independent mechanisms were also applied by Lkb1 to promote T reg cell suppressor function. AMPK-induced fatty acid oxidation is a critical metabolic feature of T reg cells [53] . To our surprise, AMPK activation is not dramatically altered in Lkb1-deficient T reg cells, and T reg cell-specific deletion of both AMPK1α and AMPK2α does not cause T reg cell abonrmality and immune disturbance, suggesting that Lkb1 does not control T reg cells by promoting AMPK activity in steady-state conditions. Lkb1 has been previously shown to promote thymocytes development, maintain survival and proliferation of peripheral T cells and restrain peripheral conventional T-cell activation and proinflammatory cytokine production [15] , [16] , [54] (we got similar results in certain experiments after inducing Lkb1 deletion in conventional T cells from ERT2 Cre Lkb1 f/f mice, Supplementary Fig. 7f,g ). Here, we find that Lkb1 maintains the lineage identity of T reg cells through mechanisms involving the regulation of NF-κB/STAT4 and TGF-β signallings ( Fig. 8 ). NF-κB/STAT4 and TGF-β signallings are separately controlled by Lkb1 ( Supplementary Fig. 7h–j ), suggesting a function of Lkb1 in setting up the optimal activation thresholds of multiple intracellular signallings in T reg cells. Furthermore, the upregulation of Lkb1 protein by TCR signalling in T reg but not in conventional T cells indicates a specific regulation of Lkb1 expression required for preserving the T reg cell lineage. Future studies will determine whether and how the environmental cues change Lkb1 in T reg cells to affect their stability/function under physiological and pathological conditions, and whether Lkb1 can be targeted to treat T reg -cell-related immune diseases. Mice All animals were maintained in specific pathogen-free barrier facilities and were used in accordance with protocols approved by the institutional animal care and user committee at the Institute of Hematology, Chinese Academy of Medical Sciences. C57BL/6, CD45.1 + , Lkb1 f/f , AMPKα1 f/f , AMPKα2 f/f , Tgfbr2 f/f , ERT2 Cre , Foxp3 YFP-Cre ( Foxp3 Cre ), Rosa26 YFP and Rag1 −/− mice were purchased from Jackson Laboratories. All mice had been backcrossed with C57BL/6 mice for at least 7 generations. Lkb1 f/f , AMPKα1 f/f , AMPKα2 f/f , Tgfbr2 f/f mice were crossed with Foxp3 Cre mice to generate Foxp3 Cre Lkb1 f/f , Foxp3 Cre AMPKα1 f/f AMPKα2 f/f and Foxp3 Cre Tgfbr2 f/f mice, respectively. Foxp3 Cre/+ Lkb1 f/f mice were crossed with Rosa26 YFP mice to generate Foxp3 Cre Lkb1 f/f Rosa26 YFP mice. Lkb1 f/f mice were crossed with ERT2 Cre and Rosa26 YFP mice to generate ERT2 Cre Lkb1 f/f Rosa26 YFP mice. Sample size for various animal experiments was chosen based on prior data generated in the laboratory, and no mice were excluded from experiments. The details of mice age and sex are provided in the figure legends. Cell purification and flow cytometry Single-cell suspensions were prepared from spleen and peripheral lymph nodes for staining or cell purification. CD4 + T cells and CD11c + DCs were purified with Dynabeads Untouched Mouse CD4 Cells Kits (Invitrogen, 11415D) or CD11c MicroBeads (Miltenyi Biotec, 130-108-338), respectively. Indicated T-cell populations were sorted from purified CD4 + T cells with FACSAria III (BD Biosciences), and the sorted populations were >98% pure unless otherwise specified. Flow cytometry of cell surface molecules was performed as previously described [55] , and the antibody ( Supplementary Data 5 ) was diluted as the instructions of the manufacturers suggested. Intracellular staining of Foxp3, cytokines (spleen cells were stimulated with phorbol myristate acetate (50 ng ml −1 ) and ionomycin (500 ng ml −1 ) for 4 h before analysis of cytokine expression in indicated populations) and other proteins were performed with Foxp3 staining kits (eBioscience, 00-5523). Intracellular staining of phosphorylated proteins was performed on cells fixed with methanol and permeabilized with Triton X-100. The antibodies were obtained from eBioscience, Biolegend, BD Biosciences, Cell Signalling Technology, R&D Systems and Invitrogen, and listed in Supplementary Data 5 . Flow cytometry data were acquired on LSR II, LSRFortessa (BD Biosciences) or FACSCanton II (BD Biosciences) and analysed with Flowjo software (Tree Star). Cell culture Sorted CD4 + YFP + T reg cells from Foxp3 Cre Lkb1 f/f and Foxp3 Cre mice were labelled with carboxyfluorescein succinimidyl ester (CFSE) Cell Proliferation Kits (Invitrogen, C34554). CFSE-labelled T reg cells were co-cultured with CD11c + cells purified from CD45.1 + mice, supplemented with indicated combinations of cytokines of recombinant murine IL-2, IL-12, IL-6 and IL-4 (all 100 ng ml −1 , PeproTech), NF-κB inhibitors sodium 4-aminosalicylate (4-ASA) or pyrrolidinedithiocarbamic acid (PDTC) or DNA methyltransferase inhibitor 5-aza-dC)in Dulbecco’s modified Eagle’s medium supplemented with 10% fetal bovine serum (Gibco) for 4 days. For inducible Lkb1 deletion, T reg cells were respectively sorted from ERT2 Cre Lkb1 f/f Rosa26 YFP and ERT2 Cre Rosa26 YFP mice and cultured for 5 days as described above, with the addition of 4-hydroxytamoxifen (1 μM, Sigma) in the culture. In other experiments, sorted T reg cells were incubated in plates precoated with anti-CD3 (2 μg ml −1 ; 145-2C11; eBioscience) and anti-CD28 (2 μg ml −1 ; 45.21; eBioscience) in the presence of IL-2 (100 ng ml −1 ) for the indicated days. CFSE profiles and Foxp3 expressions were examined by flow cytometry after culturing. In vivo T reg cell maintenance CD4 + CD25 + YFP + T reg cells were doubly sorted (>99.5% pure) from 3-week-old CD45.1 − CD45.2 + Foxp3 Cre Lkb1 f/f and CD45.1 + CD45.2 + Foxp3 Cre mice, and 2 × 10 5 of each type of cells were mixed with 4 × 10 5 CD4 + CD25 − CD44 low CD62L high T n cells sorted fromCD45.1 + CD45.2 − mice and transferred into the Rag1 −/− mice by intraperitoneal injection. The recipient mice were analysed 3 weeks after transfer. In vitro T reg cell suppression CD4 + CD25 − CD44 low CD62L high T n cells sorted from CD45.1 + mice were labelled with CFSE and used as responder cells (T resp ). T resp cells (5 × 10 4 ) were cultured for 72 h with DCs (1 × 10 5 ) and soluble anti-CD3 (2 μg ml −1 ) in the presence or absence of the indicated numbers of CD4 + YFP + T reg cells sorted from Foxp3 Cre Lkb1 f/f or Foxp3 Cre mice. Foxp3 gene methylation assay Genomic DNA from sorted cells was bisulfite converted with EZ DNA Methylation-Direct kits according to the manufacturer’s protocol (Epigentek, P-1026-050). Methylation-specific PCR primers (listed in Supplementary Data 2 ) were used for amplification of the promoter and intron 1 of Foxp3 (corresponding to Foxp3 conserved noncoding sequence 2). PCR products were subcloned into pGEM-T Easy vectors (Promega) and sequenced. Western blot CD4 + YFP + T reg cells and CD4 + YFP − conventional T cells were sorted from Foxp3 Cre and Foxp3 Cre Lkb1 f/f mice and treated as indicated, and then cells were lysed and western blot was carried out as previously described [55] with antibodies to Lkb1 (D60C5, Cell Signalling Technology), phosphorylated AMPK (40H9, Cell Signalling Technology), IKKβ (2C8, Cell Signalling Technology), phosphorylated IKKα/β (16A6, Cell Signalling Technology), phosphorylated IκBα (14D4, Cell Signalling Technology), phospho-NF-κB p65 (93H1, Cell Signalling Technology), NF-κB p65 (D14E12, Cell Signalling Technology), STAT4 (C46B10, Cell Signalling Technology), AMPKα (D63G4, Cell Signalling Technology), phospho-Acetyl-CoA Carboxylase (D7D11, Cell Signalling Technology), phospho-STAT4 (Abcam), TGF-βR2 (Abcam) and GAPDH (D16H11, Cell Signalling Technology). Microarray and quantitative real-time PCR CD4 + YFP + T reg cells were sorted from spleen and lymph nodes of mice for RNA extraction with Trizol reagent (Invitrogen). Total RNA was reverse transcribed, amplified, labelled and hybridized to Mouse Genome 2.0 arrays (Affymetrix). Microarray data sets were analysed with Agilent Genespring GS 11 software. RNA of different samples was obtained in the same manner as in microarray analysis, and real-time PCR was performed with SYBR Green PCR Master Mix (ABI) as previously described [55] . The sequences of the primer pairs used are listed in Supplementary Data 2 . DNA binding ELISA TransAM Flexi kits (Active Motif, 40098) were used to test the activity of Smad transcription factors according to the manufacturer’s protocol. Briefly, nuclear extract from stimulated T reg cells sorted from Foxp3 Cre and Foxp3 Cre Lkb1 f/f mice were mixed with biotinylated oligos (listed in Supplementary Data 2 ) recognized by transcription factors of interest, and incubated in a streptavidin-coated plate. After washing, primary antibodies specific for the bound transcription factor and horseradish peroxidase-conjugated secondary antibodies were subsequently added, and transcription factor binding activities were quantified using a microplate reader (Synergy H4, BioTek). Co-immunoprecipitation Sorted wild-type CD4 + YFP + T reg cells were expanded in plates coated with anti-CD3 (2 μg ml −1 ) and anti-CD28 (2 μg ml −1 ) in the presence of IL-2 (100 ng ml −1 ) for 5 days and collected. Cell lysis was prepared using Co-immunoprecipitation kits according to the manufacturer’s protocol (Sigma, FLAGITP1), and incubated with antibodies against Dnmt1 (60B1220.1, Abcam), Dnmt3a (Abcam) and protein G agarose (Cell Signalling Technology). Immunoprecipitated proteins were detected as described above with antibodies against STAT4 (C46B10, Cell Signalling Technology) and STAT5 (Cell Signalling Technology). Chromatin immunoprecipitation ChIP assays were performed using the ChIP kits (Active Motif, 53040) according to the manufacturer’s protocol. Precipitated DNA and input DNA were assessed by real-time PCR using primers listed in Supplementary Data 2 . Retroviral transduction TGF-βR2 cDNA was subcloned into the retroviral vector pMYs-IRES-RFP. Retroviruses were produced by transfection of the Plat-E cells with polyethylenimin. T reg cells (YFP + ) were cultured in plates coated with anti-CD3 and anti-CD28 transduced in virus-containing media supplemented with polybrene by centrifuging for 1 h at 500 RCF. After 24 h, cells were expanded and then RFP + YFP + cells were sorted before further analysis. The Plat-E cell line was provided by the Cell Resource Center, Institute of Hematology and Hospital of Blood Diseases, Chinese Academy of Medical Sciences/Peking Union Medical College. The Cell Resource Center confirmed the species origin with PCR and checked free of mycoplasma contamination by PCR and culture. Histopathology Skins, lungs, livers and stomachs were removed from 3–4-week-old mice. Samples were formalin fixed, paraffin embedded and stained with haematoxylin and eosin before tissue histology. Photomicrographs were taken at × 10 or × 20 magnifications. Statistics An unpaired two-tailed Student’s t -test (for two group comparisons) or a two-way analysis of variance (for more than two group comparisons) were performed using Prism (GraphPad) to calculate statistical significance of the difference in mean values and P values. A P value of <0.05 was considered statistically significant. * P <0.05; ** P <0.01. No specific randomization or blinding protocols were used. Data availability The data that support the findings of this study are available from the corresponding author on reasonable request. The microarray data have been deposited in the Gene Expression Omnibus under accession GSE97840. How to cite this article: Wu, D. et al . Lkb1 maintains T reg cell lineage identity. Nat. Commun. 8 , 15876 doi: 10.1038/ncomms15876 (2017). Publisher’s note: Springer Nature remains neutral with regard to jurisdictional claims in published maps and institutional affiliations.